The novel tumour suppressor Madm regulates stem cell competition in theDrosophilatestis Stem cell competition has emerged as a mechanism for selecting fit stem cells/progenitors and controlling tumourigenesis. However, little is known about the underlying molecular mechanism. Here we identify Mlf1-adaptor molecule (Madm), a novel tumour suppressor that regulates the competition between germline stem cells (GSCs) and somatic cyst stem cells (CySCs) for niche occupancy. Madm knockdown results in overexpression of the EGF receptor ligand vein ( vn ), which further activates EGF receptor signalling and integrin expression non-cell autonomously in CySCs to promote their overproliferation and ability to outcompete GSCs for niche occupancy. Conversely, expressing a constitutively activated form of the Drosophila JAK kinase ( hop Tum−l ) promotes Madm nuclear translocation, and suppresses vn and integrin expression in CySCs that allows GSCs to outcompete CySCs for niche occupancy and promotes GSC tumour formation. Tumour suppressor-mediated stem cell competition presented here could be a mechanism of tumour initiation in mammals. Animal tissues and organs are generated and maintained by stem cells, which generate most of the cell types that form an organ during development. These stem cells maintain tissue homoeostasis by supplying new cells to replace dying or damaged ones in adult animals. Recent studies suggest that Mother Nature selects the fittest stem cells for tissue development and homoeostasis through stem cell competition [1] , [2] , [3] , [4] , [5] , [6] , [7] . Stem cell competition has also been shown to be a mechanism for both tumour suppression [4] and tumour initiation [1] , [8] . However, little is known about the underlying molecular mechanism. Drosophila testis germline stem cells provide one of the best genetic systems for studying stem cell niche interactions at the cellular and molecular levels [2] , [9] , [10] , [11] , [12] , [13] , [14] , [15] , [16] , [17] , [18] , [19] , [20] , [21] , [22] , [23] , [24] , [25] , [26] , [27] , [28] , [29] , [30] , [31] , [32] , [33] . At the tip of the Drosophila testis (apex) is a germinal proliferation centre, which contains the germline stem cells (GSCs) and somatic stem cells (CySCs) that maintain spermatogenesis ( Fig. 1a ) [34] , [35] , [36] . Each GSC is encysted by two CySCs. Both the GSCs and CySCs anchor to a group of 12 non-dividing somatic cells, called the ‘hub’ [37] , through cell-adhesion molecules [31] , [38] . The hub defines the stem cell niche by expressing the growth factor Unpaired (Upd), which is the ligand that activates the JAK-STAT pathway in adjacent GSCs and CySCs to regulate their self-renewal. The ratio of GSCs to CySCs in a wild-type testis niche is 1:2 and is precisely coordinated by differentially regulating JAK-STAT signalling levels in the two different stem cell types [2] , [25] . In addition, several other signalling pathways regulate the behaviour of these two stem cells at the testis niche [20] , [21] , [39] , [40] , [41] , [42] , [43] . 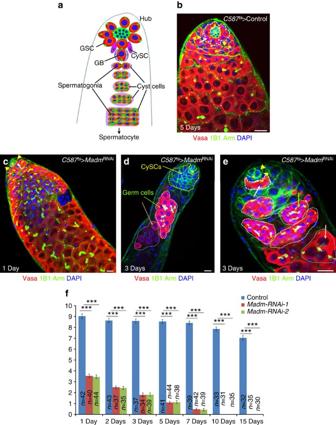Figure 1: Madm functions in CySC to regulate GSC maintenance. (a) A schematic diagram ofDrosophilaadult testis. GSCs and GBs (gonialblasts) contain the spherical spectrosomes (green dots), while spermatogonia and spermatocytes contain branched fusomes (green lines). GSCs are encysted by two CySCs (magenta). GBs and other germ cells (red) are encapsulated by cyst cells (lavender). (b–e) The confocal section of the testis apex fromC587ts>control (b), andC587ts>MadmRNAi−1(BL31644;c–e) males after shifting the temperature from 18° to 29 °C for 1 to 15 days as adult flies. In control testis (b, 5 days at 29 °C,n=41) contain a rosette of GSCs around the hub (white dotted lines with one GSC is highlighted by an arrow), and CySCs are located away from the hub (yellow arrowhead). InC587ts>MadmRNAitestes (c, 1 day,n=40; (d,e), 3 days,n=39), the number of GSCs are gradually lost from the niche and differentiated (highlighted by white dotted lines ind,e), and CySCs moved into the niche (highlighted by yellow dotted lines ind). The testes were stained with antibodies against Vasa (red, marks all germ cells including GSCs), 1B1 (green, marks spherical spectrosomes and branched fusomes), Arm (green, hub cells at the tip). DAPI (blue) stains nuclei. Asterisks indicate hub cells. White arrows near hub indicate GSC. Green arrows (ind,e) and orange arrow (d,e) away from hub with white dotted lines indicate spermatogonial cells and spermatocytes, respectively. (f) A bar graph showing the number of GSCs per testis inC587ts>control,C587ts>MadmRNAi−1(BL31644) andC587ts>MadmRNAi−2(v27346) flies. Flies were cultured from 1 to 15 days at 29 °C before staining with antibodies against Vasa, 1B1 and Arm. Statistical significance determined by Student’st-test, ***P<0.0001. All values are mean±s.e.m. Scale bar, 10 μm (b–e). Figure 1: Madm functions in CySC to regulate GSC maintenance. ( a ) A schematic diagram of Drosophila adult testis. GSCs and GBs (gonialblasts) contain the spherical spectrosomes (green dots), while spermatogonia and spermatocytes contain branched fusomes (green lines). GSCs are encysted by two CySCs (magenta). GBs and other germ cells (red) are encapsulated by cyst cells (lavender). ( b – e ) The confocal section of the testis apex from C587 ts > control ( b ), and C587 ts >Madm RNAi−1 (BL31644; c – e ) males after shifting the temperature from 18° to 29 °C for 1 to 15 days as adult flies. In control testis ( b , 5 days at 29 °C, n =41) contain a rosette of GSCs around the hub (white dotted lines with one GSC is highlighted by an arrow), and CySCs are located away from the hub (yellow arrowhead). In C587 ts >Madm RNAi testes ( c , 1 day, n =40; ( d , e ), 3 days, n =39), the number of GSCs are gradually lost from the niche and differentiated (highlighted by white dotted lines in d , e ), and CySCs moved into the niche (highlighted by yellow dotted lines in d ). The testes were stained with antibodies against Vasa (red, marks all germ cells including GSCs), 1B1 (green, marks spherical spectrosomes and branched fusomes), Arm (green, hub cells at the tip). DAPI (blue) stains nuclei. Asterisks indicate hub cells. White arrows near hub indicate GSC. Green arrows (in d , e ) and orange arrow ( d , e ) away from hub with white dotted lines indicate spermatogonial cells and spermatocytes, respectively. ( f ) A bar graph showing the number of GSCs per testis in C587 ts >control, C587 ts >Madm RNAi−1 (BL31644) and C587 ts >Madm RNAi−2 (v27346) flies. Flies were cultured from 1 to 15 days at 29 °C before staining with antibodies against Vasa, 1B1 and Arm. Statistical significance determined by Student’s t -test, *** P <0.0001. All values are mean±s.e.m. Scale bar, 10 μm ( b – e ). Full size image In a genetic screen for mutations that regulate male GSC fates, we identified Mlf1-adaptor molecule (Madm) [44] , [45] . Myeloid leukaemia factor 1 (Mlf1) is an oncogene and is originally described by a translocation between Mlf1 on chromosome 3 and nucleophosmin ( NPM ) on chromosome 5, which yields the oncogene NPM-MLF1 (ref. 46 ). Madm and 14-3-3ζ were identified as binding partners of Mlf1 in a yeast two-hybrid screen [45] . The expression of exogenous Mlf1 potentiated M1 maturation, while ectopic expression of Madm in M1 myeloid cells suppressed cytokine-induced differentiation. The opposing effects of Madm and Mlf1 on M1 cell differentiation suggest that Madm may function as a tumour suppressor. In humans, Madm was also named a nuclear receptor binding protein 1 (NRBP1) (ref. 47 ). Just as H37N21.1 ( NRBP1 ) knockdown cooperates with gain-of-function mutations in let-60 ( Ras ) to regulate vulval formation in Caenorhabditis elegans , NRBP1 knockdown cooperates with a constitutively activated form of Ras ( Ras V12 ) in the transformation of mammalian cells in culture [48] . Somatic loss of Nrbp1 in mice results in tumourigenesis, with haematological and intestinal tumours predominating. The NRBP1 protein is downregulated in a wide variety of human tumours, and survival data analysis indicates that low expression correlates with poor prognosis. These data together suggest that NRBP1 is a conserved regulator of cell fate and plays an important role in tumour suppression [48] . In this study, we show that Madm is specifically expressed in CySCs and coordinates with the JAK-STAT and EGFR signal transduction pathways to regulate stem cell competition in the Drosophila testis. Madm functions in CySCs to guide GSCs-CySCs competition To identify new stem cell regulators in the Drosophila testis, we carried out a screen in which a collection of transgenic RNAi lines [49] , [50] , [51] were crossed with act-Gal4; tub-Gal80 ts flies (referred to as Act ts ). act- Gal4 is ubiquitously expressed in the Drosophila testis ( Supplementary Fig. 1a–c ). The adult flies were shifted to the restrictive temperature (29 °C) from 18 °C and cultured for different times. The flies were then dissected, stained and examined for GSCs under confocal microscopy. One of the first few genes identified in this screen was Madm . Madm knockdown by transgenic RNAi ( Madm RNAi , BL31644) resulted in a dramatic decrease of GSCs in the testes compared with that of wild-type flies ( Supplementary Fig. 1d–g ). Knockdown of genes by dsRNAs often produce false-positive phenotypes because of off-target effects [52] . We ruled out the possibility of false-positive effects and confirmed the Madm phenotype with three other transgenic RNAi lines (v27346, BL41599 and BL42529) generated from independent sequences [49] , [51] ( Supplementary Fig. 1h,i ). To further understand the function of Madm in the germline or in the soma, we knocked down Madm by cell-type-specific Gal4s and UAS-Madm RNAi transgenic fly lines. We found that depleting Madm in germ cell lineage using nanos ( nos ) -Gal4 ( Nos > Madm RNAi ; Supplementary Fig. 1j ), and in the hub cells using unpaired ( upd ) -Gal4 ( Upd > Madm RNAi ; Supplementary Fig. 1k ) resulted in no obvious phenotype. We also generated negatively marked GSC clones of wild-type or Madm [44] flies using the FLP/FRT mosaic analysis technique [53] and found that Madm is not required in GSCs for their maintenance ( Supplementary Fig. 2a–c ). These data together suggest that Madm is not required in the germ cell lineage and hub cells. We further knocked down Madm in the CySC lineage using C587-Gal4 (refs 14 , 15 , 30 ; C587 ts > Madm RNAi ; Fig. 1b–e ) and found that the GSCs, then spermatogonia and finally spermatocytes were lost over time at 29 °C ( Fig. 1c–f and Supplementary Fig. 3a–h ) similar to the phenotypes of Act ts > Madm RNAi flies ( Supplementary Fig. 1d–g,i ), suggesting that Madm functions in the CySC lineage to regulate GSC maintenance. Further, dying GSCs were not detected in wild-type and Madm RNAi testes, and similar numbers of dying spermatogonial cysts were detected in both control and Madm RNAi testes ( Supplementary Fig. 4a–c ). In the Drosophila testis, GSCs and CySCs share the same niches. We further investigated CySCs in Madm knockdown testes by examining the expression of the zinc-finger homeodomain-1 (Zfh-1) protein, which marks CySCs and their immediate cyst cell daughters [19] ( Fig. 2a–c ). In the wild-type testes, the nuclei of Zfh-1-positive CySCs are farther from the hub than the nuclei of GSCs ( Fig. 2a , arrowhead). In the C587 ts > Madm RNAi testes, after shifting to the restrictive temperature, the Zfh-1-positive CySCs gradually moved into the niches and pushed the GSCs out ( Fig. 2b,c , arrowhead) and the number of Zfh-1-positive cells were significantly (Student’s t -test, P <0.0001) increased over time ( Fig. 2d ). Therefore, the normal function of Madm is to prevent CySCs from outcompeting GSCs for niche occupancy. 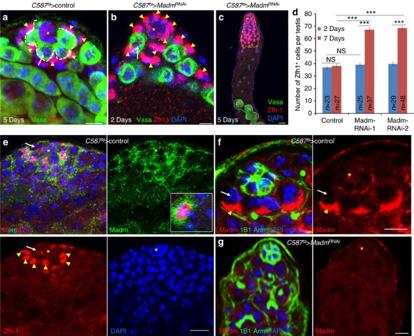Figure 2: Madm functions in CySCs to prevent CySCs from outcompeting GSCs for niche occupancy. (a–c) A confocal section of the testis apex containingC587ts>control (a) andC587ts>MadmRNAi(BL31644) (b, 2 days,n=25;c, 5 days,n=30) males after shifting the temperature from 18oto 29 °C for 2, 5 and 7 days as adult flies. The testes were stained with antibodies against Vasa (green, marks all germ cells including GSCs), Zfh-1 (red, marks CySCs and their immediate cyst cell daughters). DAPI (blue) stains nuclei. (d) A bar graph showing the number of Zfh-1+ cells per testis inC587ts>control, andC587ts>MadmRNAi−1(BL31644) andC587ts>MadmRNAi−2(v27346) flies at 2 and 7 days at 29 °C. Statistical significance determined by Student’st-test, ***P<0.0001; NS indicates not significant (P>0.05). All values are mean±s.e.m. (e–g) The testes ofC587ts>control (e) were stained with Zfh-1 (red) and Madm (green), highlighted in inset a co-stained of Zfh-1 and Madm. The testes ofC587ts>control (f) andC587ts>MadmRNAi−1(g) were stained with Madm (red), 1B1 and Arm (green), DAPI (blue). *indicate hub cells. GSCs are highlighted by white arrows and white dotted lines near hub cells inaandb, and by white arrows ineandf. Differentiated germ cells (away from the hub) incare highlighted by white dotted line (green arrow). CySCs are highlighted by arrowhead (yellow) ina,b,e,f. Yellow dotted line inchighlighted Zfh-1-positive cells. Scale bar, 10 μm (a–c,e–g). Figure 2: Madm functions in CySCs to prevent CySCs from outcompeting GSCs for niche occupancy. ( a – c ) A confocal section of the testis apex containing C587 ts >control ( a ) and C587 ts >Madm RNAi (BL31644) ( b , 2 days, n =25; c , 5 days, n =30) males after shifting the temperature from 18 o to 29 °C for 2, 5 and 7 days as adult flies. The testes were stained with antibodies against Vasa (green, marks all germ cells including GSCs), Zfh-1 (red, marks CySCs and their immediate cyst cell daughters). DAPI (blue) stains nuclei. ( d ) A bar graph showing the number of Zfh-1+ cells per testis in C587 ts > control, and C587 ts >Madm RNAi−1 (BL31644) and C587 ts >Madm RNAi−2 (v27346) flies at 2 and 7 days at 29 °C. Statistical significance determined by Student’s t -test, *** P <0.0001; NS indicates not significant ( P >0.05). All values are mean±s.e.m. ( e – g ) The testes of C587 ts > control ( e ) were stained with Zfh-1 (red) and Madm (green), highlighted in inset a co-stained of Zfh-1 and Madm. The testes of C587 ts > control ( f ) and C587 ts >Madm RNAi−1 ( g ) were stained with Madm (red), 1B1 and Arm (green), DAPI (blue). *indicate hub cells. GSCs are highlighted by white arrows and white dotted lines near hub cells in a and b , and by white arrows in e and f . Differentiated germ cells (away from the hub) in c are highlighted by white dotted line (green arrow). CySCs are highlighted by arrowhead (yellow) in a , b , e , f . Yellow dotted line in c highlighted Zfh-1-positive cells. Scale bar, 10 μm ( a – c , e – g ). Full size image Using antibodies to Madm [44] , we detected Madm expression in the somatic cells of the wild-type testes, particularly in CySC cytoplasm ( Fig. 2e,f ); while the expression of Madm was markedly reduced in the C587 ts > Madm RNAi testes ( Fig. 2g ), suggesting that Madm protein expression was effectively knocked down in the C587 ts > Madm RNAi testes. These data together suggest that Madm functions in CySCs to regulate CySCs and GSCs competition for niche occupancy. The outcompeted GSCs became differentiated rather than died We further investigated the fate of the outcompeted (loser) GSCs. First, we found that flies that had been kept in 29 °C for 3 days lacked GSCs but contained spermatogonia ( Supplementary Fig. 3c,d,h ), indicating that the outcompeted GSCs possibly became differentiated. Second, we examined cell death with TUNEL labelling of the C587 ts > Madm RNAi flies after culturing at 29 °C for 3 or 6 days and did not find any significant (Student’s t -test, P >0.05) increase of GSC death in comparison with that of the C587 ts >control flies ( Supplementary Fig. 4a–c ). Third, we wondered whether testes from Madm RNAi flies lost the GSCs at 29 °C ( Fig. 1c–f and Supplementary Fig. 3a–h ) could restore them after recovery at 18 °C. It has been demonstrated that differentiating spermatogonial cysts revert to stem cell identity when signalling is restored [10] . We fed bromodeoxyuridine to flies that had been kept in 29 °C for 3 days. These flies lacked GSCs, but contained spermatogonia ( Supplementary Fig. 3h ). Labelled CySCs were detected near the hub (arrowhead), while spermatogonial cysts (4, 8 and 16 cells) were detected away from the hub before recovery ( Supplementary Fig. 5a,b ). However, after 2 days of recovery at 18 °C, breakdown of spermatogonial cysts were detected and 14.15% of testes regained labelled GSCs ( Supplementary Fig. 5c,h ). After 4 days of recovery, 47.3% of testes regained labelled GSCs ( Supplementary Fig. 5d,e,h ). We compared the percentage of testes containing any GSCs before and after recovery, and found that after 2 days of recovery only 14.15% of testes contained any GSCs; however, 84.2% of testes contained GSCs after 6 days of recovery at 18 °C ( Supplementary Fig. 5f–h ). These data together suggest that the outcompeted GSCs became differentiated and can revert back to GSCs when the Madm activity is restored. Madm non-cell autonomously directs CySC-GSC competition To further examine the function of Madm in CySCs, we generated LacZ ( arm-lacZ )-negative CySC clones of wild-type or Madm [44] flies using the FLP/FRT mosaic analysis technique [53] and analyzed the phenotypes 3 and 12 days after clone induction (ACI) ( Fig. 3a,b and Supplementary Fig. 6a ). We uncovered a unique role of Madm in CySCs. Both wild-type and Madm mutant testes initially contain only a few LacZ-negative and Zfh-1-positive CySCs ( Fig. 3a , and Supplementary Fig. 6a ) at 3 days ACI. However, LacZ-positive and Zfh-1-positive CySCs were significantly increased and occupied the niche in the Madm mutant testes ( Fig. 3b and Supplementary Fig. 6a ), while both LacZ-negative and LacZ-positive CySCs in wild-type testes remained relatively constant at 12 days ACI [2] ( Supplementary Fig. 6a ). We also generated GFP positively marked CySC clones of wild-type or Madm flies using the mosaic analysis with a repressible cell marker (MARCM) technique [54] and analyzed CySC lineages 7 days ACI ( Fig. 3c–d ). Consistent with our previous mosaic analysis results, we found that the GFP-negative and Zfh-1-positive CySCs were significantly (Student’s t -test, P <0.0001) increased and occupied the niche in the Madm mutant testes ( Fig. 3e–h and Supplementary Fig. 6b,c ) compared with those in the wild-type testes ( Fig. 3c,d and Supplementary Fig. 6c ). Further, by staining testes with either wild-type or Madm mutant MARCM clones with GFP and Vasa, we found two unique phenotypes: (i) GFP-positive CySCs directly attaching to hub cells in Madm mutant testes while such cells locating outside GSCs in wild-type testes and (ii) only one Vasa-positive GSC left at the niche in the Madm mutant testes while normal number (5–9) of GSCs at the niche in the wild-type testes (compare Supplementary Fig. 6e–g with Supplementary Fig. 6d ). These analyses together suggest that CySCs have pushed GSCs away from the niche. We further examined the mitotic index in wild-type or C587 ts > Madm RNAi testes ( Supplementary Fig. 6h–j ) by staining with anti-phospho-Histone H3 (pH3) and found that the pH3-positive somatic cells were significantly (Student’s t -test, P <0.0001) increased in the C587 ts > Madm RNAi testes ( Supplementary Fig. 6i,j ) compared with those in the wild-type testes ( Supplementary Fig. 6h,j ). These data together suggest that Madm non-cell autonomously regulates CySC proliferation and the ability of CySCs to outcompete GSC for niche occupancy. 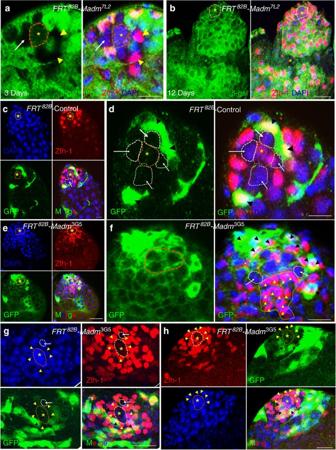Figure 3: Madm functions in CySC non-cell autonomously and regulates the competition between GSCs and CySCs. (a,b) Confocal sections through the apex of the testes containingFRT82B-Madm7L2clones at 3 days ACI (a,n=45) and 12 days ACI (b,n=52). The testes were stained with the Zfh-1 (red), β-galactosidase (green), and DAPI (blue). TheFRT82B-Madm7L2CySC clones are β-galactosidase (green) negative and Zfh-1 (red) positive. β-galactosidase negative CySCs clones are highlighted by yellow arrowhead (a,b). (c–h) GFP+veclones were generated in the testes of wild-type control (FRT82B-PiM;c,d,n=56) orFRT82B-Madm3G5(e–h,n=62) flies using the MARCM technique, and were stained at 7 days ACI with GFP (green), Zfh-1 (red) and DAPI (blue). GFP-positive CySCs clones are highlighted by black arrowheads (c–h). GFP-negative CySCs clones are highlighted by yellow arrowheads (e–h). Green arrow ineindicates differentiated germ cells. Asterisks with orange dotted lines indicate hub cells. GSCs are highlighted by white arrows and white dotted lines near hub cells. Scale bar, 10 μm (a–h). Figure 3: Madm functions in CySC non-cell autonomously and regulates the competition between GSCs and CySCs. ( a , b ) Confocal sections through the apex of the testes containing FRT 82B - Madm 7L2 clones at 3 days ACI (a, n =45) and 12 days ACI (b, n =52). The testes were stained with the Zfh-1 (red), β-galactosidase (green), and DAPI (blue). The FRT 82B -Madm 7L2 CySC clones are β-galactosidase (green) negative and Zfh-1 (red) positive. β-galactosidase negative CySCs clones are highlighted by yellow arrowhead ( a , b ). ( c – h ) GFP +ve clones were generated in the testes of wild-type control ( FRT 82B -PiM ; c , d , n =56) or FRT 82B -Madm 3G5 ( e – h , n =62) flies using the MARCM technique, and were stained at 7 days ACI with GFP (green), Zfh-1 (red) and DAPI (blue). GFP-positive CySCs clones are highlighted by black arrowheads ( c – h ). GFP-negative CySCs clones are highlighted by yellow arrowheads ( e – h ). Green arrow in e indicates differentiated germ cells. Asterisks with orange dotted lines indicate hub cells. GSCs are highlighted by white arrows and white dotted lines near hub cells. Scale bar, 10 μm ( a – h ). Full size image Madm non-cell autonomously regulates integrin and p-dERK It was reported that SOCS36E suppresses JAK-STAT signalling specifically in the CySCs, preventing them from displacing neighbouring GSCs, by upregulating the adhesion protein integrin [2] , [25] . The function of Madm is somehow similar to that of SOCS36E. The expression of Stat92E is regulated by JAK-STAT signalling and the level of Stat92E protein reflects JAK-STAT signalling activity [55] . To investigate the function of Madm on JAK-STAT signalling, we examined Stat92E protein expression in wild-type and Madm knockdown testes ( C587 ts > Madm RNAi ) ( Supplementary Fig. 7a–d ). In wild-type testes, Stat92E is specifically enriched in GSCs, while CySCs, hub cells and all differentiated cells express little Stat92E, indicating that GSCs normally have higher JAK-STAT signalling than that of CySCs ( Supplementary Fig. 7a,e ). In Madm knockdown testes ( C587 ts > Madm RNAi ; Supplementary Fig. 7b–d ), CySCs and hub cells have elevated levels of Stat92E ( Supplementary Fig. 7e ). This result suggests that Madm , functioning similarly to SOCS36E, normally attenuates JAK-STAT signalling in CySCs and hub cells to maintain the appropriate balance of the two stem cell lineages in the niche. We further examined the expression of the common β-subunit of position-specific integrins (βPS-integrin) in wild-type and Madm knockdown testes ( C587 ts > Madm RNAi ; Supplementary Fig. 8a–f ). The βPS-integrin level is significantly (Student’s t -test, P <0.0001) higher in Madm knockdown testes ( Supplementary Figs 8c,d,g ) than in wild-type testes ( Supplementary Fig. 8a,b,g ), particularly at the CySC–hub interface ( Supplementary Fig. 8c,f ). We also examined the expression of βPS-integrin together with DE-cadherin (mark hub cells) and found that integrin is not incorporated in hub cells, but rather highly expressed at the hub-CySC interface in Madm knockdown testes ( Supplementary Fig. 8f ). The number and appearance of hub cells were unaffected in Madm knockdown testes as compared with wild-type testes ( Supplementary Fig. 8e,f ; Control: 22.83±0.41, n =12, versus Madm RNAi : 24.14±0.55, n =14, hub cells per testis, P >0.05). This result indicates that Madm may regulate stem cell competition by controlling integrin expression. To further test this hypothesis, we examined the genetic interaction between Madm and rhea , an integrin-binding cytoskeletal linker that is essential for integrin-mediated adhesion [56] . Removing one copy of rhea did not cause GSC loss, but it did significantly (one-way analysis of variance, P <0.0001) suppress the phenotype of Madm knockdown testes ( C587 ts > Madm RNAi ; Supplementary Fig. 9 ). These results suggest that Madm normally prevents CySCs from outcompeting GSCs for niche occupancy via an integrin-mediated mechanism. We also examined βPS-integrin expression in GFP positively marked CySC MARCM clones of wild-type or Madm flies ( Fig. 4a,b ). Surprisingly, we found that the βPS-integrin level was significantly (Student’s t -test, P <0.0001) higher in both GFP-positive Madm mutant CySCs and GFP-negative wild-type CySCs in the Madm testes ( Fig. 4b,c ) than the level in the wild-type testes ( Fig. 4a,c ), particularly at the CySC–hub interface, indicating that Madm regulates integrin expression non-cell autonomously. 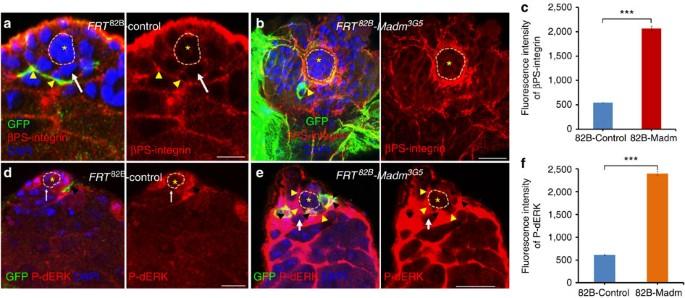Figure 4: Madm regulates integrin and p-dERK expression non-cell autonomously. (a,b) GFP+veclones were generated in the testes of wild-type control (FRT82B-PiM(a,n=27) andFRT82B-Madm3G5(b,n=32) clones at 3 days ACI. βPS-integrin expression is markedly increased inMadm3G5testes at the CySCs–hub interface compared with wild-type control testes. The testes were immunostained with βPS-integrin (red), GFP (green) and DAPI (blue). GSCs are highlighted by white arrows. GFP-positive clones are highlighted by arrowhead (yellow,a,b). (c) A bar graph showing the quantitation of fluorescence intensity of βPS-integrin inFRT82B-PiMandFRT82B-Madm3G5testes at the CySC–hub interface. (d,e) GFP-positive clones were generated in the testes of wild-type control (FRT82B-PiM(d,n=35) andFRT82B-Madm3G5(e,n=37) clones at 3 days ACI. p-dERK expression is markedly increased inFRT82B-Madm3G5testes in both GFP-positive cells and GFP−vecells compared with wild-type control testes. The testes were immunostained with p-dERK (red), GFP (green) and DAPI (blue). GFP-positive clones are highlighted by arrowhead (black,d,e) and GFP-positive cells are highlighted by arrowhead (yellow,d,e). GSCs are highlighted by white arrows. (f) A bar graph showing the quantitation of fluorescence intensity of p-dERK inFRT82B-PiMandFRT82B-Madm3G5testes. Asterisks with orange dotted lines indicate hub cells. All values are mean±s.e.m. Statistical significance determined by Student’st-test, ***P<0.0001. Scale bar, 10 μm (a,b,d,e). Figure 4: Madm regulates integrin and p-dERK expression non-cell autonomously. ( a , b ) GFP +ve clones were generated in the testes of wild-type control ( FRT 82B -PiM ( a , n =27) and FRT 82B -Madm 3G5 ( b , n =32) clones at 3 days ACI. βPS-integrin expression is markedly increased in Madm 3G5 testes at the CySCs–hub interface compared with wild-type control testes. The testes were immunostained with βPS-integrin (red), GFP (green) and DAPI (blue). GSCs are highlighted by white arrows. GFP-positive clones are highlighted by arrowhead (yellow, a , b ). ( c ) A bar graph showing the quantitation of fluorescence intensity of βPS-integrin in FRT 82B -PiM and FRT 82B -Madm 3G5 testes at the CySC–hub interface. ( d , e ) GFP-positive clones were generated in the testes of wild-type control ( FRT 82B -PiM ( d , n =35) and FRT 82B -Madm 3G5 ( e , n =37) clones at 3 days ACI. p-dERK expression is markedly increased in FRT 82B -Madm 3G5 testes in both GFP-positive cells and GFP −ve cells compared with wild-type control testes. The testes were immunostained with p-dERK (red), GFP (green) and DAPI (blue). GFP-positive clones are highlighted by arrowhead (black, d , e ) and GFP-positive cells are highlighted by arrowhead (yellow, d , e ). GSCs are highlighted by white arrows. ( f ) A bar graph showing the quantitation of fluorescence intensity of p-dERK in FRT 82B -PiM and FRT 82B -Madm 3G5 testes. Asterisks with orange dotted lines indicate hub cells. All values are mean±s.e.m. Statistical significance determined by Student’s t -test, *** P <0.0001. Scale bar, 10 μm ( a , b , d , e ). Full size image Similarly, we examined the expression of phosphorylated Drosophila ERK (p-dERK) in GFP positively marked CySC MARCM clones of wild-type or Madm testes ( Fig. 4d,e ). Again, we were surprised to find that the p-dERK level was significantly (Student’s t -test, P <0.0001) higher in both GFP-positive Madm mutant CySCs and GFP-negative wild-type CySCs in the Madm testes ( Fig. 4e,f ) than the level in the wild-type testes ( Fig. 4d,f ), indicating that Madm regulates p-dERK expression non-cell autonomously. We further tested the genetic interaction between Madm and its components in the EGFR signal transduction pathway and found that reducing the dosage of several components in the EGFR pathway significantly (one-way analysis of variance, P <0.0001) suppressed the phenotype of the Madm knockdown testes ( C587 ts > Madm RNAi ; Supplementary Fig. 9 ). These results suggest that the EGFR signal transduction pathway functions either downstream or in parallel to Madm in regulating the competition between CySCs and GSCs for niche occupancy. Mlf1 and Madm play opposite roles in stem cell competition Madm and the oncogene Mlf1 have opposing functions in regulating M1 cell differentiation [45] . We examined the function of Mlf1 in regulating stem cell competition by examining the expression of Zfh-1 and Stat92E in C587 ts >Mlf1 testes. In the wild-type testes, the nuclei of Zfh-1-positive CySCs are farther from the hub than the nuclei of GSCs ( Supplementary Fig. 10a ). In both C587 ts > Madm RNAi ( Supplementary Fig. 10b ) and C587 ts >Mlf1 testes ( Supplementary Fig. 10c ), after shifting to the restrictive temperature, the Zfh-1-positive CySCs gradually moved into the niches and pushed GSCs out ( Supplementary Fig. 10b,c ). We also found that CySCs and hub cells had elevated levels of Stat92E in C587 ts >Mlf1 testes compared with control testes ( Supplementary Fig. 10d–f ), similar to those in C587 ts > Madm RNAi testes ( Supplementary Fig. 7b–e ). These data together suggest that the oncogene Mlf1 and tumour suppressor Madm play opposite roles in regulating stem cell competition in the Drosophila testis. The Ras-Raf pathway regulates CySCs–GSCs competition The data described above indicate that both the JAK-STAT and EGFR signal transduction pathways may function downstream of Madm in regulating stem cell competition through integrin. However, hop Tum − l (the activated JAK kinase) overexpression in CySCs ( C587 ts > hop Tum − l ) did not produce the stem cell competition phenotype rather than GSC tumours [19] , [57] ( Fig. 5b , compare with Fig. 5a ). To examine the function of the EGFR signal transduction in regulating the competition between CySCs and GSCs for niche occupancy, we expressed a constitutively activated form of Ras ( Ras V12 ) and a gain-of-function mutant form of Raf ( Raf gof ) in somatic cells ( C587 ts > Ras V12 , Fig. 5c and Supplementary Fig. 11a ; and C587 ts > Raf gof ; Supplementary Fig. 11c ). Elevation of EGFR signalling through Ras V12 or Raf gof expression in somatic cells resulted in CySC overproliferation and CySCs outcompeting GSCs for niche occupancy ( Fig. 5c , Supplementary Figs 11a,c ), similar to what was seen in phenotypes of knocking down Madm in somatic cells ( Figs 1c–e and 2b,c ). We further expressed hop Tum − l with Ras V12 ( C587 ts > hop Tum − l /Ras V12 ; Fig. 5d and Supplementary Fig. 11b ) or hop Tum − l with Raf gof ( C587 ts > hop Tum − l /Raf gof ; Supplementary Fig. 11d ) in somatic cells and found that the testes expressing the double transgenes had phenotypes similar to the testes expressing Ras V12 or Raf gof alone. These results suggest that the EGFR/Ras/Raf/ERK pathway functions either downstream or in parallel of the JAK signal transduction pathway in regulating the ability of CySCs to outcompete GSCs for niche occupancy. We also examined the expression of βPS-integrin in the testes with GFP-positive marked CySC MARCM clones of control ( Fig. 5e,f ), Ras V12 ( Fig. 5g,h ) and hop Tum − l ( Fig. 5i,j ) or in C587 ts > hop Tum − l ( Supplementary Fig. 11e ) and C587 ts > Ras V12 ( Supplementary Fig. 11f ) testes. We found that only Ras V12 induced βPS-integrin expression in these experiments ( Fig. 5h,k ), which was consistent with the above functions of hop Tum − l and Ras V12 in regulating competition between CySCs and GSCs for niche occupancy. 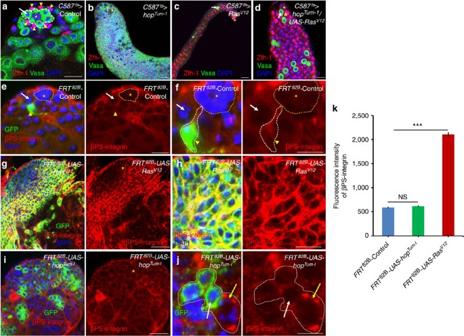Figure 5: The Ras, rather than the JAK (Hop), regulates the competition between CySCs and GSCs for niche occupancy. (a–d) Confocal sections of the testes containingC587ts>Control (a,n=26),C587ts>hopTum−l(b,n=25),C587ts>RasV12(c,n=20), andC587ts>hopTum−l/RasV12(d,n=27). The testes were cultured for 6 days at 29 °C before they were immunostained with Zfh-1 (red), Vasa (green) and DAPI (blue). GSCs are highlighted by white arrows and white dotted lines near hub cells (a–d). CySCs are highlighted by arrowhead (yellow,a–d). (e–k) GFP+veclones were generated in the testes ofFRT82B-PiM(e,f),FRT82B-UAS-RasV12(g,h;n=45) andFRT82B-UAS-hopTum−l(i,j;n=37) flies using the MARCM technique and were stained at 6 days ACI with antibodies against GFP (green) and βPS-integrin (red). DAPI (blue) stained nuclei. InFRT82B-UAS-RasV12testes integrin is highly elevated in GFP+veCySC clones (g,h); however, inFRT82B-UAS-hopTum−ltestes, integrin is weakly expressed (i,j). GSCs are highlighted by white arrows. (k) A bar graph showing the quantitation of fluorescence intensity of βPS-integrin inFRT82B-PiM,FRT82B-UAS-RasV12andFRT82B-UAS-hopTum−ltestes. *indicate hub cells. All values are mean±s.e.m. Statistical significance determined by Student’st-test, ***P<0.0001. Scale bar, 10 μm (a–j). Figure 5: The Ras, rather than the JAK (Hop), regulates the competition between CySCs and GSCs for niche occupancy. ( a – d ) Confocal sections of the testes containing C587 ts > Control ( a , n =26), C587 ts >hop Tum − l ( b , n =25), C587 ts >Ras V12 ( c , n =20), and C587 ts >hop Tum − l /Ras V12 ( d , n =27). The testes were cultured for 6 days at 29 °C before they were immunostained with Zfh-1 (red), Vasa (green) and DAPI (blue). GSCs are highlighted by white arrows and white dotted lines near hub cells ( a – d ). CySCs are highlighted by arrowhead (yellow, a – d ). ( e – k ) GFP +ve clones were generated in the testes of FRT 82B -PiM ( e , f ), FRT 82B -UAS-Ras V12 ( g , h ; n =45) and FRT 82B -UAS-hop Tum − l ( i , j ; n =37) flies using the MARCM technique and were stained at 6 days ACI with antibodies against GFP (green) and βPS-integrin (red). DAPI (blue) stained nuclei. In FRT 82B -UAS-Ras V12 testes integrin is highly elevated in GFP +ve CySC clones ( g , h ); however, in FRT 82B -UAS-hop Tum − l testes, integrin is weakly expressed ( i , j ). GSCs are highlighted by white arrows. ( k ) A bar graph showing the quantitation of fluorescence intensity of βPS-integrin in FRT 82B -PiM , FRT 82B -UAS-Ras V12 and FRT 82B -UAS-hop Tum − l testes. *indicate hub cells. All values are mean±s.e.m. Statistical significance determined by Student’s t -test, *** P <0.0001. Scale bar, 10 μm ( a – j ). Full size image These data together suggest that the EGFR/Ras/Raf/ERK pathway may function downstream of the JAK-STAT signal transduction pathway in regulating the competition between CySCs and GSCs for niche occupancy by controlling integrin expression. The JAK pathway regulates nuclear translocation of Madm To explore the relationship between Madm and the JAK-STAT signal transduction pathway, we compared Madm protein expression in wild-type ( Fig. 6a,b ) and C587 ts > hop Tum − l testes (compare Fig. 6c,d with Fig. 6a,b ), and found that most Madm translocated into the nuclei in the C587 ts > hop Tum−l flies ( Fig. 6c,d ), while the Madm protein was mostly localized to the cytoplasm in wild-type flies ( Fig. 6a,b ). We further found that expressing C587 ts > hop Tum − l / Madm RNAi produced a phenotype similar to expressing C587 ts > Madm RNAi ( Fig. 6e ), suggesting that hop Tum − l regulates stem cell competition through Madm. 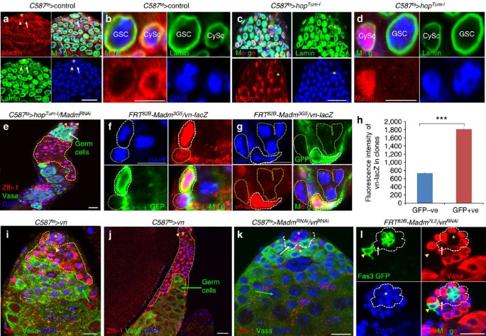Figure 6: JAK signaling regulates the nuclear translocation of Madm, and Madm negatively regulates the EGFR/Ras/ERK signaling pathway by repressingvnexpression. (a–d) The testes ofC587ts>Control (6 days,a,b;n=15),C587ts>hopTum−l(6 days;c,d;n=32) were immunostained with the Madm (red), Lamin (red) and DAPI (blue). *indicate hub cells (a,c). GSC is highlighted by white arrows and CySCs are highlighted by yellow arrowhead (a,c). (e) The testes ofC587ts>hopTum−l/MadmRNAi(6 days,n=25). Testes were cultured for 7 days at 29 °C before they were immunostained with Zfh-1 (red), Vasa (green) and DAPI (blue). (f,g) The testes ofFRT82B-Madm3G5/vn-lacZ(n=33) were immunostained with β-galactosidase (vn-lacZ-red), GFP (green) and DAPI (blue).vnexpression is markedly increased in GFP-positiveMadmmutant CySCs (white dotted lines) compared with GFP-negative CySCs (yellow dotted lines). (h) A bar graph showing the quantitation of fluorescence intensity ofvn-LacZinFRT82B-Madmmutant clones. (i–k). Confocal sections of the testes containingC587ts>vn(i(70%) andj(30%);n=32); andC587ts>MadmRNAi/vnRNAi(k,n=30). The testes were cultured for 7 days at 29 °C before they were immunostained with Zfh-1 (red), Vasa (green) and DAPI (blue). (l) The testes ofFRT82B-Madm7L2/vnRNAi(n=22) were immunostained 4 days ACI with GFP (green, yellow arrowhead), Fas3 (green, hub cells), Vasa (red) and DAPI (blue).vnknockdown in GFP-marked MARCM CySC clones ofMadmmutant significantly (Student’st-test,P<0.0001) suppress the phenotypes associated withMadmknockdown. Green arrows indicate differentiated germ cells (e,i,j). Yellow arrowhead indicate CySCs (e,i–l). GSC are highlighted by white arrows (white dotted lines,k,l). Yellow dotted lines indicate Zfh-1-positive cells (e,i,j). *indicate hub cells. All values are mean±s.e.m. Statistical significance determined by Student’st-test, ***P<0.0001. Scale bar, 10 μm (a–h). Figure 6: JAK signaling regulates the nuclear translocation of Madm, and Madm negatively regulates the EGFR/Ras/ERK signaling pathway by repressing vn expression. ( a – d ) The testes of C587 ts > Control (6 days, a , b ; n =15), C587 ts >hop Tum − l (6 days; c , d ; n =32) were immunostained with the Madm (red), Lamin (red) and DAPI (blue). *indicate hub cells ( a , c ). GSC is highlighted by white arrows and CySCs are highlighted by yellow arrowhead ( a , c ). ( e ) The testes of C587 ts >hop Tum − l /Madm RNAi (6 days, n =25). Testes were cultured for 7 days at 29 °C before they were immunostained with Zfh-1 (red), Vasa (green) and DAPI (blue). ( f , g ) The testes of FRT 82B -Madm 3G5 /vn-lacZ ( n =33) were immunostained with β-galactosidase ( vn - lacZ -red), GFP (green) and DAPI (blue). vn expression is markedly increased in GFP-positive Madm mutant CySCs (white dotted lines) compared with GFP-negative CySCs (yellow dotted lines). ( h ) A bar graph showing the quantitation of fluorescence intensity of vn-LacZ in FRT 82B -Madm mutant clones. ( i – k ). Confocal sections of the testes containing C587 ts >vn ( i (70%) and j (30%); n =32); and C587 ts >Madm RNAi /vn RNAi ( k , n =30). The testes were cultured for 7 days at 29 °C before they were immunostained with Zfh-1 (red), Vasa (green) and DAPI (blue). ( l ) The testes of FRT 82B -Madm 7L2 /vn RNAi ( n =22) were immunostained 4 days ACI with GFP (green, yellow arrowhead), Fas3 (green, hub cells), Vasa (red) and DAPI (blue). vn knockdown in GFP-marked MARCM CySC clones of Madm mutant significantly (Student’s t -test, P <0.0001) suppress the phenotypes associated with Madm knockdown. Green arrows indicate differentiated germ cells ( e , i , j ). Yellow arrowhead indicate CySCs ( e , i – l ). GSC are highlighted by white arrows (white dotted lines, k , l ). Yellow dotted lines indicate Zfh-1-positive cells ( e , i , j ). *indicate hub cells. All values are mean±s.e.m. Statistical significance determined by Student’s t -test, *** P <0.0001. Scale bar, 10 μm ( a – h ). Full size image We also examined Madm expression in C587 ts > Stat92E AC (a constitutively activated version of Stat92E) and C587 ts > Socs36E RNAi testes, and we did not find increasing nuclear translocation of Madm ( Supplementary Fig. 12a ), suggesting that Stat92E and Socs36E do not regulate Madm nuclear translocation. We further generated Socs36E RNAi MARCM clones ( Supplementary Fig. 12b–d ) and found that only GFP-positive CySCs were moved to the tip of the testes, and outcompete GSCs for niche occupancy. These data together suggest that only activated JAK ( hop Tum − l ) regulates Madm nuclear translocation, and Socs36E may function in the EGFR signal transduction pathway and regulate stem cell competition cell autonomously. Madm represses the expression of EGFR ligand vein in CySCs We further investigated the relationship between Madm and the EGFR signal transduction pathway. We demonstrated that knockdown of Madm non-cell autonomously induced p-dERK expression ( Fig. 4d–f ), and our data also suggest that the EGFR signal transduction pathway may function downstream of Madm and the JAK-STAT signal transduction pathway in regulating stem cell competition. This information indicates that Madm may regulate stem cell competition by repressing EGFR ligand expression in the testis. Spitz (Spi) and Vein (Vn) are two major ligands of EGFR [58] . We examined their gene expressions in the testes using their respective LacZ reporters. Consistent with a previous finding [59] , we found that spi is expressed in germ cells ( Supplementary Fig. 12e ); vn was mainly expressed in somatic cells, including CySCs ( Supplementary Fig. 12f ). To further investigate the relationship between Madm mutation and vn expression, we generated GFP-marked MARCM CySC clones of Madm mutant with vn-lacZ ( Fig. 6f–h ) and found that vn expression was markedly increased in GFP-positive Madm mutant CySCs compared with that in GFP-negative wild-type CySCs ( Fig. 6f–h ). We also generated the flip-out clones in the testes of hs-flp; Ay>Gal4/UAS-GFP+UAS-Madm RNAi +vn-LacZ flies and again found that vn expression was markedly increased in GFP-positive Madm RNAi CySCs compared with that in GFP-negative wild-type CySCs ( Supplementary Fig. 12g,h ). These data together suggest that Madm represses vn expression in CySCs. We further found that vn overexpression promoted the CySCs’ ability to outcompete GSCs for niche occupancy (similar to the phenotype of Madm knockdown; Fig. 6i,j ). Knockdown of vn alone in CySCs results in GSC tumour phenotypes ( Supplementary Fig. 12i ), similar to those of knockdown of Egfr ( Fig. 7a ). Co-knockdown of vn and Madm in CySCs suppressed the phenotype of Madm knockdown ( Fig. 6k ) and expression of vn RNAi in Madm mutant MARCM CySC clones restored the testes to the phenotypes of wild-type testes ( Fig. 6l , compare Fig. 6l with Supplementary Fig. 6d–g ). These data demonstrated that vn is the major downstream target of Madm . 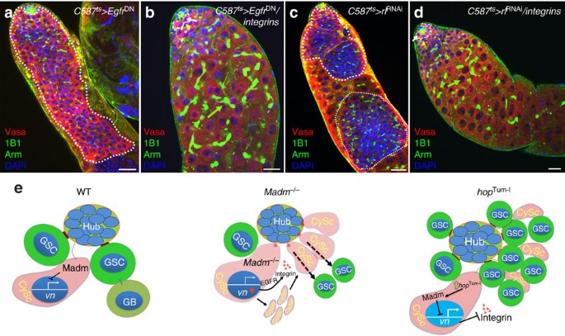Figure 7: The overexpression of integrin rescued the GSC tumour phenotypes associated with the loss of EGFR-ERK signaling and overexpression ofZfh-1. (a–d) GSCs in the testes ofC587ts>EgfrDN(a,n=22),C587ts>EgrfDN/PS1βPS (integrins)(b,n=32),C587ts>rlRNAi(c,n=30) andC587ts>rlRNAi/PS1βPS (integrins)(d,n=35). The testes were cultured for 7 days at 29 °C before they were immunostained with Vasa (red), 1B1 and Arm (green) and DAPI (blue). *indicate hub cells. GSCs are highlighted by white arrows (b,d). CySCs are highlighted by arrowhead (yellow,b,d). White dotted lines in a and c representing GSC tumour phenotype. (e) A model of how Madm regulates GSC and CySC competition inDrosophilatestis. Details are described in the text. Scale bar, 10 μm (a–d). Figure 7: The overexpression of integrin rescued the GSC tumour phenotypes associated with the loss of EGFR-ERK signaling and overexpression of Zfh-1. ( a – d ) GSCs in the testes of C587 ts >Egfr DN ( a , n =22), C587 ts >Egrf DN /PS1βPS (integrins) ( b , n =32), C587 ts >rl RNAi ( c , n =30) and C587 ts >rl RNAi /PS1βPS (integrins) ( d , n =35). The testes were cultured for 7 days at 29 °C before they were immunostained with Vasa (red), 1B1 and Arm (green) and DAPI (blue). *indicate hub cells. GSCs are highlighted by white arrows ( b , d ). CySCs are highlighted by arrowhead (yellow, b , d ). White dotted lines in a and c representing GSC tumour phenotype. ( e ) A model of how Madm regulates GSC and CySC competition in Drosophila testis. Details are described in the text. Scale bar, 10 μm ( a – d ). Full size image We also found that the expression of a constitutively activated form of EGFR ( C587 ts > λtop ; Supplementary Fig. 13a,b ) could promote the ability of CySCs to outcompete GSCs for niche occupancy and stimulate Stat92E expression in CySCs ( Supplementary Fig. 13b,c ). These data together suggest that in such a model knocking down Madm may first result in vn overexpression, which further activates the EGFR signal transduction pathway non-cell autonomously to activate Stat92E and induce integrin expression in CySCs, so that CySCs outcompete GSCs for niche occupancy. Integrin overexpression can rescue the GSC tumour phenotypes Our data described above demonstrated that the activated EGFR/Ras signal transduction pathway regulates integrin expression, and that integrin plays a pivotal role in controlling the competition between CySCs and GSCs for niche occupancy. Loss-of-function mutations in the EGFR signal transduction pathway [17] , [27] or overexpression of zfh-1 and hop Tum − l resulted in GSC tumour phenotypes [19] . We examined the function of integrin in regulating GSC tumour phenotypes associated with expressing a dominant-negative form of EGFR ( Egfr DN ; Fig. 7a ), dERK RNAi ( rl RNAi ; Fig. 7c ), or zfh-1 ( Supplementary Fig. 13d ) in somatic cells. We found that integrin overexpression could significantly (Student’s t -test, P <0.0001) rescue the GSC tumour phenotypes associated with expressing a dominant-negative form of EGFR ( EGFR DN ; Fig. 7b ), rl RNAi ( Fig. 7d ), zfh-1 ( Supplementary Fig. 13e ) and hop Tum − l ( Supplementary Fig. 14a ) in somatic cells. These data suggest that the loss of EGFR-ERK signalling and overexpression of zfh-1 and hop Tum − l may downregulate integrin expression in CySCs, which is important for allowing GSCs to outcompete CySCs for niche occupancy and in promoting GSC tumour formation. We further examined vn expression in the testes that overexpressed hop Tum − l ( C587 ts > hop Tum − l / vn-lacZ ) and found that vn expression was markedly suppressed ( Supplementary Fig. 14b in comparison with Supplementary Fig. 12f ). These data together suggest that expressing the activated JAK kinase ( hop Tum − l ) promotes Madm nuclear translocation, which further suppresses vn and integrin expression in CySCs that allows GSCs to outcompete CySCs for niche occupancy and promotes GSC tumour formation. In this study, we have shown that the novel tumour suppressor Madm regulates the competition between GSCs and CySCs for niche occupancy in the adult Drosophila testis. We found that Madm is specifically expressed in CySCs and knockdown of Madm results in the overexpression of the EGF receptor ligand vn , which further activates EGF receptor signalling and integrin expression non-cell autonomously in CySCs to promote their overproliferation and ability to outcompete GSCs for niche occupancy. Conversely, expressing a constitutively activated form of Drosophila JAK kinase ( hop Tum − l ) promotes Madm nuclear translocation and suppresses vn and integrin expression in CySCs, allowing GSCs to outcompete CySCs in niche occupancy and promoting GSC tumour formation ( Fig. 7e and Supplementary Fig. 14c ). The loss of EGFR-ERK signalling or overexpression of zfh-1 and chinmo in CySCs also resulted in GSC tumour formation [17] , [19] , [27] , [57] . We found that overexpressing integrin can significantly (Student’s t -test, P <0.0001) rescue the GSC tumour phenotypes associated with the loss of EGFR-ERK signalling and overexpression of zfh-1 and hop Tum − l . These results together suggest that the relative integrin level in CySCs determines whether GSCs or CySCs occupy the niche, while the tumour suppressor, and signal transduction pathways regulate stem cell competition and stem cell tumour formation by modulating integrin expression. In human and mouse hematopoietic stem cells (HSCs), breast and other cancer systems, integrins play important roles in regulating stemness, stem cell competition and cancer stem cell formation [60] , [61] , [62] . It was recently reported that the reduced expression of CD18 (a leukocyte integrin) leads to a cell-autonomous in vivo expansion of early quiescent short-term and long-term HSCs in mouse bone marrow [61] . Remarkably, the CD18-low HSCs are more competitive than their wild-type counterparts in the bone marrow competition assays of recipient mice. Therefore, low integrins in this case make HSCs more competitive. In many other cases, the opposite seems to be true. High expression of the α6 integrin subunit (CD49f) is a biomarker for breast and other cancer stem cells [60] . A recent publication further demonstrated that integrin α v β 3 serves as a marker/driver of carcinoma stemness that is highly resistant to receptor tyrosine kinase inhibitors such as erlotinib [62] . The integrin α v β 3 regulates tumour initiation, anchorage independence, self-renewal and erlotinib resistance by activating the KRAS-RalB-NF-κB pathway. In this study, we further revealed the molecular details of how a tumour suppressor and the signal transduction pathways of JAK and EGFR coordinately regulate stem cell competition and stem cell tumour formation by manipulating integrin expression in one type of stem cells. Stem cell competition generally involves three steps. The competitive stem cells first become more fit before they move and anchor to a special location (such as a niche) by expressing cell-adhesion molecules, and finally eliminate the outcompeted stem cells. In the mouse thymus, the ‘young’ bone marrow-derived progenitors are more fit; they move to the thymus to gain survival advantages by contacting the survival factor IL-7 and increasing the expression of intracellular pro-survival protein Bcl2. The ‘old’ thymus-resident progenitors have low survival advantages because they have low affinity to IL-7, express low levels of Bcl2, and are eliminated through apoptosis [4] . However, it is not clear what changes make the bone marrow-derived progenitors more fit and what molecules mediate the young progenitors’ move to the thymus and cause them to remain there. In p53 -deficient mice, the p53 -low hematopoietic stem and progenitor cells are more competitive (have advantages in proliferation and long-term maintenance), may be located to a special microenvironment (niche), and also induce growth arrest and senescence-related gene expression non-cell autonomously in the outcompeted p53 -high hematopoietic stem and progenitor cells by expressing an unknown secreting factor [1] , [8] . In the Drosophila ovary, the differentiation-defective bam - or bgcn -mutant GSCs are more competitive, and they invade the niche space of neighbouring wild-type GSCs by upregulating the adhesion molecule E-cadherin. The detached wild-type GSCs from the niche will go through differentiation [3] . In this case, the self-renewal-promoting BMP signal is not required in stem cell competition. However, in another study, it was found that the GSCs expressing high levels of Drosophila Myc (dMyc) were more competitive than the dMyc-low GSCs [5] . The niche-provided self-renewal factor BMP/DPP in metabolically active dMyc-high GSCs is required for stem cell competition. In the Drosophila testis, we demonstrated that the tumour suppressor Madm- deficient CySCs are more competitive. The Madm- deficient CySCs overexpress the EGF receptor ligand vn , which secretes to the intercellular fluid and activates EGF receptor signalling non-cell autonomously in CySCs to stimulate CySC proliferation and increase integrin expression. The elevated integrin gives CySCs the advantage of outcompeting GSCs for niche occupancy. The niche signal Upd may activate JAK-STAT signalling in CySCs to further enhance fitness and maintenance of CySCs. The outcompeted GSCs will leave the niche and become differentiated. Conversely, promoting Madm nuclear translocation by expressing the hop Tum − l or knocking down EGFR signalling will suppress integrin expression in CySCs, which will give GSCs the advantage of outcompeting CySCs for niche occupancy and will result in GSC tumour formation. p53 and Madm share some similarities in regulating stem cell competition. They both regulate stem cell competition non-cell autonomously. In mice, the p53 -deficient HSCs may secrete an unknown factor that non-cell autonomously promotes proliferation and long-term maintenance in the p53 -low cells and, at the same time, induces growth arrest and senescence-related gene expression in the p53 -high cells [1] , [8] . In Drosophila , our study demonstrated that Madm -deficient CySCs induce the expression of the EGFR ligand vn , which further activates EGF receptor signalling and integrin expression non-cell autonomously to promote CySC proliferation and the ability of CySCs to outcompete GSCs for niche occupancy. Furthermore, unlike what often happens in other cell competitions [63] , the outcompeted ‘loser’ stem cells were not eliminated through cell death. In the p53 case, the loser HSCs became senescent; in the Madm case, the loser GSCs became differentiated. Altogether, these data suggest that stem cell (or cancer stem cell) competition may be a fundamental mechanism of tumour formation. The knowledge gained from studying tumour suppressor-mediated stem cell competition will help to understand the unique molecular basis of tumour initiation and may be used to develop novel drug targets for advancing cancer therapy. Drosophila stocks and cultures Oregon R was used as the wild-type strain. The other fly stocks used in this study are either described in FlyBase or as otherwise specified. Nos-Gal4 ( nanosGal4VP16 ) (ref. 64 ), Act-Gal4 , tub-GAL80 ts , Act5C-GAL4.UAS-GFP , UAS-GFP.nls , UAS-mCD8-GFP hs-Flp , SM6 , hs-Flp , and tub-Gal4 FRT82B-tub-Gal80 , UAS-Ras V12 , UAS-Raf gof , Egfr F24 , UAS-Mlf1 , Egfr DN , UAS-Zfh-1 , spi-lacZ (BL10462), vn-lacZ (BL11749), UAS-GFP RNAi and Madm RNAi lines -BL31644 (Madm RNAi−1 ), BL41599, BL42529 were obtained from the Bloomington stock centre; rl RNAi (v35641), Madm RNAi−2 (v27346) and Socs36 RNAi (v51821) were obtained from Vienna Drosophila Resource Centre (VDRC); vn RNAi (10491R-2) was obtained from the National Institute of Genetics (NIG), Japan; Drk TZ160 and Ras c40b are our lab stocks; rl 698 is from Norbert Perrimon; upd-Gal4 and c587-Gal4 were provided by Ting Xie; UAS-hop Tum − l was provided by Erika Bach and Soichi Tanda ; UAS-vn was provided by Jocelyn Donaldson and Amanda Simcox; UAS-PS1 βPS ( integrins ) was provided by Kendal Broadie; rhea 6 − 66 and rhea 13 − 8 were provided by Amin Ghabrial; UAS-λtop was provided by Trudi Schupbach; FRT 82B - Madm 3G5 and FRT 82B - Madm 7L2 were provided by Hugo Stocker. Flies were raised on standard fly food at 25 °C and at 65% humidity, unless otherwise indicated. Genes and mutations that are not described in the text can be found at Flybase ( http://flybase.bio.indiana.edu ). RNAi-mediated gene depletion Male UAS-RNAi transgene flies were crossed with female virgins of genotype Nos-Gal4 , upd-Gal4 , c587-Gal4; tub-Gal80 ts ( c587 ts ) or Act-Gal4; tub-Gal80 ts ( Act ts ). The flies were cultured at 18 °C. Three- to 5-day-old adult flies with the appropriate genotype were transferred to new vials at 29 °C for 1 to 15 days before dissection. The sequences used for VDRC knockdown strains are available for each line at https://stockcenter.vdrc.at , and sequences for Bloomington knockdown strains are available for each line at http://flystocks.bio.indiana.edu . These sequences are also shown in Supplementary Note 1 . Generating mutant GSCs clones Clones of mutant GSCs were generated as previously described [31] . To generate Madm mutant GSC clones, FRT 82B /+ and FRT 82B - Madm 3G5 / Cyo or FRT 82B - Madm 7L2 / Cyo virgin females were mated with males of genotype FRT 82B - arm-lacZ / Cyo ; SM6, hs-flp/+. Genotypes used to induce mutant clones are provided in Supplementary Note 1 . One- or 2-day-old adult males carrying an arm-lacZ transgene in trans to the mutant-bearing chromosome were heat-shocked four times at 37 °C for 1 h, at intervals of 8–12 h. The males were transferred to fresh food every day at 25 °C. The testes were removed 1, 2, 4, 7 and 12 days after the first heat-shock treatment and processed for antibody staining. MARCM clonal analysis Clones of GFP-marked mutant CySCs for control ( FRT 82B -PiM/ +); and mutants ( FRT 82B -PiM/+; FRT 82B - UAS - hop Tum − l /+; FRT 82B - UAS - Ras V12 /+; UAS - Socs36E RNAi /+; FRT 82B -Madm 3G5 ; FRT 82B -Madm 7L2 ) were generated using the MARCM system [54] . Detail of genotypes used to induce MARCM clones are provided in Supplementary Note 1 . Three- or 4-day-old adult female flies were heat-shocked twice at 37 °C for 45 min, with intervals of 8–12 h. The flies were transferred to fresh food daily after the final heat shock. The testes were removed at 1, 2 or 7 days after the first heat-shock treatment and processed for antibody staining. Immunofluorescence staining and microscopy Immunofluorescence staining was performed as previously described with some modifications [31] . Briefly, the testes were dissected in 1 × PBS, transferred to 4% formaldehyde in 1 × PBS and fixed for 30 min. The testes were then washed in PBST (PBS containing 0.1% Triton X-100) for 3 times for 10 min each time and blocked with 2% goat serum in PBST for 1 h. Samples were incubated with primary antibody in 1 × PBST at 4 °C overnight. Samples were washed for three times, 10 min each time in 1 × PBST, then incubated with secondary antibody in 1 × PBST at room temperature for 2 h, washed as previously described, and mounted in VECTASHIELD with DAPI (Vector Labs). The following antisera were used: rabbit polyclonal anti-Vasa antibody (1:1,000; a gift from Ruth Lehmann), rabbit polyclonal anti-β-Gal antibody (1:1,000; Cappel), mouse monoclonal anti-β-Gal antibody (1:100; Invitrogen), mouse monoclonal anti-Hts antibody 1B1 (1:20; DSHB); rabbit anti-Madm (1: 500; a gift from Hugo Stocker), rabbit polyclonal anti-GFP antibody (1:200; Invitrogen), mouse monoclonal anti-GFP antibody (1:100; Invitrogen), rabbit polyclonal anti-phosphorylated histone H3 (pH3) antibody (1:1,000; Upstate), guinea pig polyclonal anti-Zfh-1 (1:2,000; a gift from James Skeath), rabbit polyclonal anti-Stat92E (1:500; ref. 55 ), mouse anti-βPS-integrin (1:20; DSHB), rabbit anti-p-dERK (1:200; Cell Signalling), rat anti-bromodeoxyuridine (1:50; Serotec), mouse anti-Fas3, rat anti-DE-cadherin and mouse anti-armadillo (Arm) N7A1 (1:20; DSHB). Secondary antibodies were goat anti-mouse, goat anti-guinea pig and goat anti-rabbit IgG conjugated to Alexa 488 or Alexa 568 (1:400; Invitrogen). Apoptosis was detected via TUNEL with the ApopTag Red In Situ Apoptosis Detection Kit (Chemicon International) according to the manufacturer’s instructions. DAPI (Invitrogen) and VECTASHIELD with DAPI (Vector Labs) were used to stain DNA. Confocal images were obtained by using a Zeiss LSM510 system, and were processed with Adobe Photoshop CS6. Bromodeoxyuridine Labelling We followed the protocol described by Brawley and Matunis [10] . In brief, male flies were starved for 8–10 h, and then fed 100 mM bromodeoxyuridine (Chem-Implex International) in yeast and sucrose paste with added green food colour to monitor feeding for 3 h at 29 °C. Testes were dissected and fixed immediately or allowed to recover for 2–4 days at 18 °C before dissection. Testes were fixed in 4% paraformaldehyde (in 1 × PBS) for 30 min at room temperature, then washed 3 times with 1 × PBX, and rinsed in 1 × PBS. Testes were then incubated with DNaseI (Promega) for 30 min at 37 °C before immunostaining [31] . Quantification and statistical analysis The number of GSCs/testis and CySCs/testis was counted using serial confocal reconstructions of the entire testis apex [2] . Vasa-positive cells (with spherical spectrosomes) contacting the hub were scored as GSCs. Zfh-1-positive cells contacting the hub were scored as CySCs as described by Issigonis et al. [2] , and Leatherman and Dinardo [19] . Statistical analyses of GSC and CySC numbers (mean±s.e.m.) were performed using GraphPad Prism program. Sample sizes ( n ) reported reflect the individual testis number. All experiments were performed in triplicates. P values were obtained between two groups using the Student’s t -test or between more than two groups by analysis of variance. For all statistical analysis, differences were considered to be statistically significant at values of P <0.05. To quantify the strength of fluorescence of Stat92E, βPS-integrin, p-DERK and vn-lacZ, all images were taken with the same confocal settings. For quantification, mean intensities of several individual cells attaching directly to hub cells in individual testis were measured. The fluorescence intensity was measured using an LSM5 image Browser (Zeiss). How to cite this article : Singh, S. R. et al. The novel tumour suppressor Madm regulates stem cell competition in the Drosophila testis. Nat. Commun. 7:10473 doi: 10.1038/ncomms10473 (2016).